Synthesis and X-ray characterization of 15- and 16-vertexcloso-carboranes 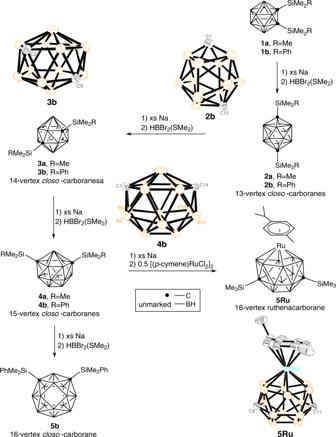Fig. 1: Synthesis of 13- to 16-vertexcloso-carboranes and 16-vertex ruthenacarborane. Synthetic route along with the molecular structures of 13-vertexcloso-carborane (2b), 14-vertexcloso-carborane (3b), 15-vertexcloso-carborane (4b), and 16-vertex ruthenacarborane (5Ru). For clarity, in the X-ray structures, all silyl moieties and hydrogen atoms have been omitted. Orange, B; grey, C. Carboranes are a class of carbon-boron molecular clusters with three-dimensional aromaticity, and inherent robustness. These endowments enable carboranes as valuable building blocks for applications ranging from functional materials to pharmaceuticals. Thus, the chemistry of carboranes has received tremendous research interest, and significant progress has been made in the past decades. However, many attempts to the synthesis of carboranes with more than 14 vertices had been unsuccessful since the report of a 14-vertex carborane in 2005. The question arises as to whether these long sought-after molecules exist. We describe in this article the synthesis and structural characterization of 15- and 16-vertex closo -carboranes as well as 16-vertex ruthenacarborane. Such a success relies on the introduction of silyl groups to both cage carbons, stabilizing the corresponding nido -carborane dianions and promoting the capitation reaction with HBBr 2 ·SMe 2. This work would shed some light on the preparation of carboranes with 17 vertices or more, and open the door for studying supercarborane chemistry. Carboranes are a class of carbon-boron molecular clusters with 3D aromaticity. They are finding a wide variety of applications as functional building blocks in the supramolecular design, medicine, catalysts, nanomaterials, and more [1] , [2] . These applications would be benefitted from higher nuclearity clusters containing large numbers of boron atoms. Thus, the chemistry of carboranes has attracted tremendous attention, particularly in the catalytic selective functionalization of carboranes [1] , [3] , [4] , [5] , [6] , [7] , [8] , [9] , [10] , [11] and polyhedral expansion for the synthesis of supercarboranes (carboranes with more than 12 vertices) [12] , [13] , [14] . In contrast to the extensively studied icosahedral o -carboranes that have dominated the carborane chemistry for over half a century [1] , [15] , [16] , has considerable progress been made in the chemistry of supercarboranes only since 2003 [12] . Such a breakthrough relied on the use of relatively weaker reducing compounds, CAd (carbon atoms-adjacent) nido -carborane dianions or arachno -carborane tetraanions [17] , as starting materials for polyhedral expansion reactions [18] , [19] . A number of 13- and 14-vertex closo -carboranes were prepared and structurally characterized [20] , [21] , [22] , [23] , [24] , [25] , [26] , [27] , [28] , [29] . They showed some unique characteristics. For example, a 13-vertex closo -carborane accepted one electron to give a stable carborane radical anion with [2 n + 3] framework electrons [30] , [31] ; it also reacted with various nucleophiles to afford the cage carbon and/or cage boron extrusion products closo -CB 11 − , nido -CB 10 − , closo -CB 10 − , and closo -C 2 B 10 , depending on the nature of the nucleophiles [32] , [33] , [34] , [35] . Insertion of a metal fragment into a 14-vertex CAd nido -carborane was successful, resulting in the isolation and structural characterization of a 15-vertex metallacarborane 1,4-(CH 2 ) 3 -7-( p -cymene)-7,1,4-RuC 2 B 12 H 12 [23] . 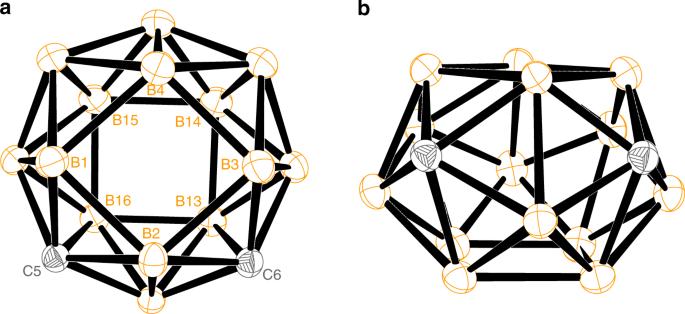Fig. 2: Molecular structure of 16-vertexcloso-carborane 5b in different view angles. aView down from the B(1)B(2)B(3)B(4) face.bView down from the C(5) and C(6) atoms. Both silyl moieties and hydrogen atoms are omitted for clarity. Orange, B; grey, C. However, the reactions of CAd [ nido -(CH 2 ) 3 C 2 B 12 H 12 ]Na 2 with haloboranes RBX 2 under different reaction conditions did not afford any 15-vertex closo -carborane, rather generated a structural isomer of CAd 14-vertex closo -carborane along with some inseparable very polar boron-containing species [23] . These results indicated that redox reaction proceeded in the system, in which nido -carborane was oxidized to the corresponding closo -species. To suppress such redox reactions and promote the capping reaction, a 14-vertex nido -carborane with lower reducing power is necessary. It was documented that silyl groups can stabilize carboanions and the stabilization is approximately additive for the number of silyl groups [36] . We then speculated that the introduction of silyl groups to both cage carbon vertices should significantly stabilize the corresponding nido -carborane dianions, so as to lower their reducing power. On the other hand, our experimental and theoretical results indicate that CAp (carbon atoms-apart) closo -carboranes are thermodynamically more stable than the corresponding CAd closo- species [37] . For instance, CAp 15-vertex carborane is calculated to be thermodynamically more stable over CAd isomer by 22.4 kcal/mol [37] . In view of the role of silyl groups and extra stability of CAp supercarboranes, we initiated a research program to prepare supercarboranes using 1,2-(R 3 Si) 2 -1,2-C 2 B 10 H 10 as starting materials. In this work, we report the synthesis and structural characterization of CAp 15- and 16-vertex closo -carboranes as well as 16-vertex ruthenacarborane. The results indicate that they are thermodynamically very stable. 15-Vertex closo -carborane Reduction of 1,2-(RMe 2 Si) 2 -1,2-C 2 B 10 H 10 [R = Me ( 1a ), Ph ( 1b )] with an excess amount of finely cut sodium metal in THF at room temperature gave presumably CAp nido -carborane salts [{7,9-(RMe 2 Si) 2 -7,9-C 2 B 10 H 10 }{Na 2 (THF) x }] [38] , [39] . Treatment of these salts with 2 equiv. of HBBr 2 ·SMe 2 in dimethoxyethane (DME) from −78 to 25 °C afforded, after column chromatographic separation, CAp 13-vertex closo -carboranes 1,12-(RMe 2 Si) 2 -1,12-C 2 B 11 H 11 [R = Me ( 2a ), Ph ( 2b )] in 20–29% isolated yields. Their 11 B NMR spectra exhibited a pattern of 1:2:1:3:3:1 ranging from δ = 15 to −17 ppm. Single-crystal X-ray analyses confirm that the cage carbons are located in 1- and 12-positions, respectively, in both 2a and 2b (Fig. 1 ). Fig. 1: Synthesis of 13- to 16-vertex closo -carboranes and 16-vertex ruthenacarborane. Synthetic route along with the molecular structures of 13-vertex closo -carborane ( 2b ), 14-vertex closo -carborane ( 3b ), 15-vertex closo -carborane ( 4b ), and 16-vertex ruthenacarborane ( 5Ru ). For clarity, in the X-ray structures, all silyl moieties and hydrogen atoms have been omitted. Orange, B; grey, C. Full size image Treatment of 2 with an excess amount of finely cut sodium metal in THF at room temperature, followed by the reaction with 3 equiv. of HBBr 2 ·SMe 2 in CH 2 Cl 2 (DCM) from −78 to 25 °C afforded, after column chromatographic separation, CAp 14-vertex closo -carboranes 2,9-(RMe 2 Si) 2 -2,9-C 2 B 12 H 12 [R = Me ( 3a ), Ph ( 3b )] in 15–20% isolated yields (Fig. 1 ). The 11 B NMR spectra of 3 exhibited a pattern of 2:4:4:2, ranging from δ = 10 to −20 ppm. Their solid-state structures were further confirmed by single-crystal X-ray analyses, showing that they adopt a bicapped hexagonal antiprismatic geometry as that of 2,9-Me 2 -2,9-C 2 B 12 H 12 [27] , with two cage carbons being located at 2- and 9-positions. Compounds 3 were treated with an excess amount of finely cut sodium metal in THF, followed by the reaction with 3 equiv. of HBBr 2 ·SMe 2 from −78 to 25 °C in CH 2 Cl 2 gave, after column chromatographic separation, 1,14-(RMe 2 Si) 2 -1,14-C 2 B 13 H 13 [R = Me ( 4a ), Ph ( 4b )] in 3–8% isolated yields (Fig. 1 ). Their 11 B NMR spectra showed a pattern of 2:4:4:1:2 spanning the range δ = 16 to −21 ppm. Single-crystal X-ray analyses show that 4b adopts a closo structure with 26 triangulated faces and 32 framework electrons. It has an approximate D 3h symmetry with a C 3 axis passing through the centers of C(1)B(2)B(3) and B(13)C(14)B(15) trigonal planes if omitting two dimethylphenylsilyl (DMPS) groups and the differentia among boron and carbon atoms. The two 6-coordinate cage carbons are located at 1-, 14-positions, respectively, which is the second stable CAp isomer predicted by DFT results [37] . There are three 7-coordinate [B(7), B(8) and B(9)], and ten 6-coordinate boron atoms. 16-Vertex ruthenacarborane Reduction of 4a with an excess amount of finely cut sodium metal in THF at room temperature, followed by interaction with 0.5 equiv. of [( p -cymene)RuCl 2 ] 2 in THF from −30 to 25 °C afforded, after column chromatographic separation, a 16-vertex ruthenacarborane 9,11-(Me 3 Si) 2 -1-( p -cymene)-1,9,11-RuC 2 B 13 H 13 ( 5Ru ) in 38% isolated yield as yellow crystals. Its 11 B NMR spectrum exhibited a 2:2:2:1:4:2 pattern in the range δ = 0.1 to −28.2 ppm, which was very different from that of 4a . Single-crystal X-ray analyses revealed that 5Ru adopts a closo structure with 26 triangular and one rhombus faces, in which the Ru atom is η 6 -bonded to a six-membered B 6 ring with an average Ru-B distance of 2.274(3) Å (Fig. 1 ) [40] , [41] . This measured value is very close to that of 2.247(3) Å in 1,4-(CH 2 ) 3 -7-( p -cymene)-7,1,4-RuC 2 B 12 H 12 [23] . The two 6-coordinate cage carbons are located in 9- and 11-positions, respectively. Careful examination of the X-ray structures of 4b and 5Ru clearly indicated that significant cage rearrangement occurred during the reaction. A DSD (diamond-square-diamond) mechanism may be involved in such a skeletal rearrangement [42] . 16-Vertex closo -carborane Treatment of 4b with an excess amount of finely cut sodium in THF at room temperature for 3 days, followed by reaction with 3 equiv. of HBBr 2 ·SMe 2 in CH 2 Cl 2 afforded, after column chromatographic separation, a CAp 16-vertex closo -carborane 5b in 26% isolated yield as colorless crystals (Fig. 1 ). It is stable in air and soluble in common organic solvents such as n -hexane, acetone, CH 2 Cl 2 , and CHCl 3 . Attempts to prepare closo -C 2 B 14 H 16 by removing two silyl groups from 5b were not successful. The 11 B NMR spectrum of 5b displayed a pattern of 1:4:4:3:2 spanning the range δ = 14.3 to −18.3 ppm. Its solid-state structure was confirmed by single-crystal X-ray analyses (Fig. 2 ). Compound 5b adopts a closo structure with 34 framework electrons, 24 triangular and two rhombus faces, in which the two 6-coordinate cage carbons are located in the 5, 6-positions, respectively. If omitting two DMPS groups and the differentia among boron and carbon atoms, 5b has an approximate D 4d symmetry with a C 4 axis passing through the centers of B(1)B(2)B(3)B(4) and B(13)B(14)B(15)B(16) faces (Fig. 2 a). Such a geometry is predicted to be the third most stable isomer by DFT calculation [37] . It could also be viewed as a square-crown-square type of structure with two cage carbons located on the crown (Fig. 2b ). Fig. 2: Molecular structure of 16-vertex closo -carborane 5b in different view angles. a View down from the B(1)B(2)B(3)B(4) face. b View down from the C(5) and C(6) atoms. Both silyl moieties and hydrogen atoms are omitted for clarity. Orange, B; grey, C. Full size image It has been well documented that closo -carboranes/ closo -polyhedral boranes are three-dimensional aromatic molecules, which have electrons delocalized through a set of orbitals tangential to the polyhedral surface [43] , [44] . The structural features of 4b and 5b were confirmed by density functional theory (DFT) calculations at the B3LYP level of theory (see computational details in the Supplementary Information and cartesian coordinates in Supplementary Data 1 and 2 ). The HOMO (highest occupied molecular orbital) is composed of the contribution of the π orbitals of the phenyl rings from the SiMe 2 Ph groups (see Supplementary Figs. 8 and 9 ). The LUMO (lowest unoccupied molecular orbitals) exhibits anti-bonding characters of cage tangential orbitals. 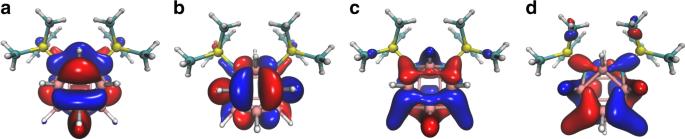Fig. 3: Selected molecular orbitals of 16-vertexcloso-carborane 5b calculated at the B3LYP/6-31G(d,p) level of theory. aLUMO + 1.bLUMO.cHOMO-4.dHOMO-5. Figure 3 shows the LUMO, LUMO + 1, HOMO-4, and HOMO-5 orbitals of 5b . Fig. 3: Selected molecular orbitals of 16-vertex closo -carborane 5b calculated at the B3LYP/6-31G(d,p) level of theory. a LUMO + 1. b LUMO. c HOMO-4. d HOMO-5. Full size image In summary, we have prepared and fully characterized 15- and 16-vertex closo -carboranes as well as 16-vertex ruthenacarborane. The results indicate that they are thermodynamically very stable. Such a success relies on the introduction of silyls onto the two cage carbons, stabilizing the corresponding nido -carborane dianions, and thus facilitating the capitation reaction. Following this strategy, if silyl groups would be introduced to cage boron atoms, it is anticipated that carboranes with 17 vertices or more would be prepared in the future as they are calculated to be thermodynamically more stable than 13- and 15-vertex closo- carboranes [37] . On the other hand, it is further anticipated that these superclusters may find applications in coordination chemistry/materials science in view of the recent development in this field [45] , [46] , [47] , [48] . The synthetic protocol and the characterization of compounds 1a – 4a , 1b – 5b , and 5Ru can be found in the Supplementary Information.